Greater efficiency of photosynthetic carbon fixation due to single amino-acid substitution The C4-photosynthetic carbon cycle is an elaborated addition to the classical C3-photosynthetic pathway, which improves solar conversion efficiency. The key enzyme in this pathway, phosphoenolpyruvate carboxylase, has evolved from an ancestral non-photosynthetic C3 phosphoenolpyruvate carboxylase. During evolution, C4 phosphoenolpyruvate carboxylase has increased its kinetic efficiency and reduced its sensitivity towards the feedback inhibitors malate and aspartate. An open question is the molecular basis of the shift in inhibitor tolerance. Here we show that a single-point mutation is sufficient to account for the drastic differences between the inhibitor tolerances of C3 and C4 phosphoenolpyruvate carboxylases. We solved high-resolution X-ray crystal structures of a C3 phosphoenolpyruvate carboxylase and a closely related C4 phosphoenolpyruvate carboxylase. The comparison of both structures revealed that Arg884 supports tight inhibitor binding in the C3-type enzyme. In the C4 phosphoenolpyruvate carboxylase isoform, this arginine is replaced by glycine. The substitution reduces inhibitor affinity and enables the enzyme to participate in the C4 photosynthesis pathway. Based on the type of CO 2 assimilation, plants can be divided into three photosynthetic types: the C3-type, the C4-type and the Crassulacean Acid Metabolism [1] . In the classical C3-photosynthetic pathway, the primary CO 2 fixation is catalysed by the enzyme ribulose-1,5-bisphosphate carboxylase/oxygenase (RuBisCO) resulting in the formation of the three-carbon compound 3-phosphoglycerate. However, in high temperature conditions RuBisCO is prone to energy loss by a process called photorespiration [2] . In C4 plants, this energy loss is minimized by an additional CO 2 concentrating mechanism. This new mechanism evolved to adapt to stress factors such as heat, high light and salinity in combination with low CO 2 availability in recent geological history [3] . The relevant key enzyme of this pathway, phosphoenolpyruvate (PEP) carboxylase (PEPC), catalyses the HCO 3 -dependent carboxylation of PEP to form the four-carbon molecule oxaloacetate [1] . Subsequent to the carboxylation reaction, oxaloacetate is reduced to malate or transaminated to aspartate. Both C4 molecules form a reservoir pool for the malic enzyme or PEP carboxykinase. These enzymes generate a high CO 2 concentration at the active site of RuBisCO. Thereby RuBisCO’s oxygenase activity is reduced and the photosynthetic efficiency is increased in terms of use of water, nitrogen and other mineral nutrients for the production of valuable biomass [3] . For the CO 2 concentration mechanism, it is necessary to spatially separate the primary CO 2 fixation by PEPC and the CO 2 release to RuBisCO. Most C4 plants realize this by a characteristic anatomical feature, the Kranz anatomy, which spatially separates RuBisCO in the bundle-sheath cells from the initial site of CO 2 assimilation in the mesophyll cells [4] . Other mechanisms of compartmentation of the photosynthetic enzymes within cells have also been reported [5] . Another crucial step in the evolution of the C4 pathway is the recruitment of enzymes such as PEPC and the malic enzyme, which are required for initial CO 2 fixation and CO 2 release, respectively [6] . The predecessors for these C4 enzymes are enzymes from C3 plants and are involved in non-photosynthetic metabolic processes. However, the C4-type enzymes have distinctly different kinetic and regulatory properties. For instance, C4 PEPC shows tenfold larger substrate saturation constants for PEP [7] than the C3 PEPC and higher tolerance towards feedback inhibition by the C4-dicarboxylic acids malate and aspartate [8] . Previous studies imply that the acquisition of this enhanced tolerance towards feedback inhibition is an essential achievement in the evolution of C4 PEPC from the C3 ancestor [9] . A prime example of the evolution of C4 photosynthesis is found in the genus Flaveria (yellowtops) in the Asteraceae family. It includes species that perform C3 photosynthesis (for example, F. pringlei ), C4 photosynthesis (for example, F. trinervia ) as well as C3–C4 intermediate metabolism (for example, F. pubescens ) [10] . All species within the genus are closely related and therefore ideal model organisms to pinpoint the key mutations that led from C3 to C4 photosynthesis [11] . In the case of PEPC, the C4 isoform from F. trinervia (encoded by the ppcA gene) and its corresponding non-photosynthetic C3 isoform, the orthologous ppcA gene of F. pringlei [12] , share 94% amino-acid (aa) identity. But along with differences in location and function, they show distinct differences in their kinetic and regulatory properties [8] . The C3 ppcA gene of F. pringlei is assumed to be similar to the PEPC that was ancestral to the C3 and the C4 PEPCs in the genus Flaveria [13] . The differences in kinetic efficiency have been addressed by reciprocal domain swapping and site-specific mutagenesis experiments. The increased PEP saturation kinetics of the C4 isoform depends on a single aa (Ser774) [14] . Less is known about the regulatory motif conferring the high malate/aspartate tolerance of C4 PEPC, which is imperative for the C4 cycle. Mutagenesis experiments indicate that the malate tolerance is largely mediated by the carboxy-terminal region of C4 PEPC (aa 645–966) [8] , and residues Arg641, Lys829, Arg888 and Asn964 ( Flaveria numbering) together have been identified as the malate-binding motif in the crystal structure of a C4-type PEPC from maize [15] . Mutagenesis of residues Lys829 and Arg888 was shown to completely disrupt the feedback inhibitor-binding site and results in enzymes with highly reduced malate sensitivity [16] . However, as this malate-binding motif is also found in the C3-type ortholog, these residues cannot account for the different feedback inhibitor sensitivity of C3- and C4-type PEPCs. Despite intensive studies [17] , [18] , no specific residue or motif was identified to account for the increased malate/aspartate tolerance of the photosynthetic C4 PEPC in comparison with the C3 PEPC isoform. As sequence analysis and mutagenesis studies failed to elucidate the molecular basis for malate/aspartate tolerance, we determined the crystal structures of PEPC isoforms from the C4 plant F. trinervia (2.5 Å) as well as from the C3 plant F. pringlei (2.7 Å) in their inhibited T-conformation. Our structures help to define the molecular adaptation that occurred when the housekeeping C3 isoform mutated to the photosynthetic C4 PEPC. X-ray crystallography Crystal structures of PEPC from Zea mays (maize), a representative C4 isoform, and from Escherichia coli , a non-photosynthetic C3 PEPC catalysing typical housekeeping functions, are known [17] , [19] . However, the low level of sequence similarity (40%) [17] in these enzymes impeded the correlation of structural differences to C4-related features. Furthermore, the fact that the C4 structure was crystallized in the activated R-state and the C3 structure in the inhibited T-state may have resulted in the high level of backbone variation in multiple regions of the monomers ( Fig. 1a ). In contrast, any differences detected in the substrate site or the inhibitor-binding pocket of the PEPC isoforms from F. pringlei and F. trinervia can be attributed to a C3/C4-specific function. We crystallized PEPC from F. pringlei and F. trinervia with the inhibitor aspartate. We chose aspartate because malate and aspartate are equivalent feedback inhibitors and the addition of malate impeded crystal growth. 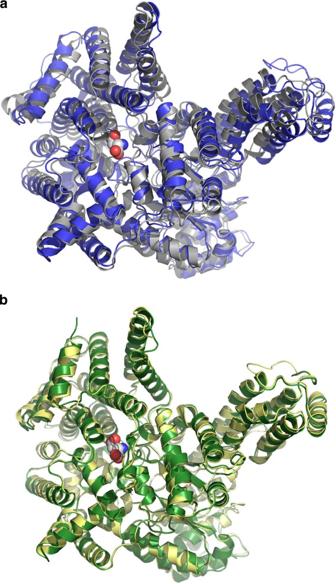Figure 1: Structural comparison of C3 PEPC and C4 PEPC monomers. (a) Overlay of PEPC fromE. coli(C3-type, grey)17andZ. mays(C4-type, blue)17. The calculated root-mean-square deviaton (r.m.s.d.) of both monomers is 2.0 Å. (b) Superposition of PEPC fromF. pringlei(C3-type, green) andF. trinervia(C4-type, yellow). TheFlaveriaPEPCs have a high overall topological similarity with a r.m.s.d. of 0.4 Å. Structures are shown as ribbons with the aspartate/malate-binding site on top. The bound inhibitors are shown as spheres representing van der Waals radii. The crystallographic data and the refinement statistics are shown in Table 1 . The Ramachandran plot of the refined C3 PEPC structure showed that the backbone conformation of 97.2% of the residues lies in the favoured region, 2.5% in the allowed region and 0.3% in the outlier region. The C4 PEPC structure has 97.9% favoured residues, 1.8% allowed residues and 0.2% outliers. Figure 1: Structural comparison of C3 PEPC and C4 PEPC monomers. ( a ) Overlay of PEPC from E. coli (C3-type, grey) [17] and Z. mays (C4-type, blue) [17] . The calculated root-mean-square deviaton (r.m.s.d.) of both monomers is 2.0 Å. ( b ) Superposition of PEPC from F. pringlei (C3-type, green) and F. trinervia (C4-type, yellow). The Flaveria PEPCs have a high overall topological similarity with a r.m.s.d. of 0.4 Å. Structures are shown as ribbons with the aspartate/malate-binding site on top. The bound inhibitors are shown as spheres representing van der Waals radii. Full size image Table 1 Data collection and refinement statistics. Full size table The structural superposition of the PEPCs from F. pringlei and F. trinervia ( Fig. 1b ) confirms the high level of structural similarity, which is also reflected in the low backbone root-mean-square deviation of 0.4 Å. A closer look at the inhibitor-binding site reveals that residue 884, which is located close to the feedback inhibitor-binding site, differs in the C3 and the C4 isoforms ( Fig. 2 and corresponding stereo views in Fig. 3 ). The C3 PEPC isoform from F. pringlei has an arginine that is involved in inhibitor binding and functions as a molecular clamp tightening the inhibitory aspartate molecule in the binding pocket. In the C4 PEPC isoform from F. trinervia this arginine is replaced by glycine. The substitution reduces the number of protein–inhibitor interactions and provides more steric space for the inhibitor to dissociate from the binding pocket ( Fig. 4 ). This important change is caused by a single-point mutation changing codon AGA to GGA. Thus, the structural comparison between the two Flaveria PEPC isoforms provides a unique way to analyse the function of these enzymes. 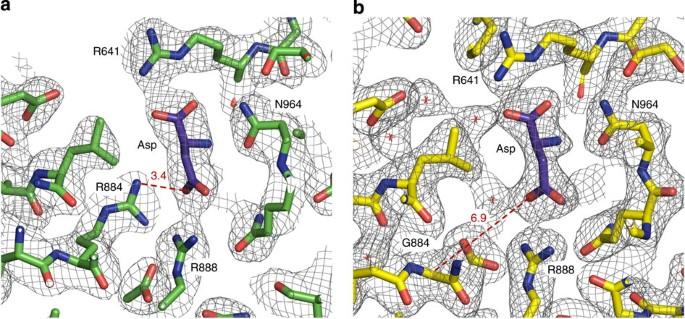Figure 2: Comparison of the inhibitor-binding sites. (a) C3 PEPC fromF. pringlei.(b) C4 PEPC fromF. trinervia. Arg884 in C3 PEPC functions as a clamp by providing an additional hydrogen bond for inhibitor binding, while Gly884 in C4 PEPC is more than 6 Å away from the inhibitor. Structures and 2Fo−Fcelectron densities at 1.2σof the malate/aspartate-binding pockets. Figure 2: Comparison of the inhibitor-binding sites. ( a ) C3 PEPC from F. pringlei. ( b ) C4 PEPC from F. trinervia . Arg884 in C3 PEPC functions as a clamp by providing an additional hydrogen bond for inhibitor binding, while Gly884 in C4 PEPC is more than 6 Å away from the inhibitor. Structures and 2 F o − F c electron densities at 1.2 σ of the malate/aspartate-binding pockets. 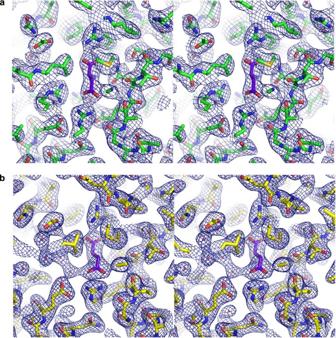Figure 3: Electron density maps and final model structures. (a) C3 PEPC fromF. pringlei,(b) C4 PEPC fromF. trinervia. Shown are the refined 2Fo−Fcelectron density maps around the inhibitor-binding sites. The maps are contoured at 1.2σ, whereσrepresents the root mean square of the density fluctuation of the unit cell. The model structures are shown as sticks. Carbon atoms are coloured green, yellow and purple forF. pringleiPEPC,F. trinveriaPEPC and the inhibitor Asp, respectively. Nitrogen atoms are coloured blue, oxygens red and sulphurs yellow. Full size image Figure 3: Electron density maps and final model structures. ( a ) C3 PEPC from F. pringlei, ( b ) C4 PEPC from F. trinervia . Shown are the refined 2 F o − F c electron density maps around the inhibitor-binding sites. The maps are contoured at 1.2 σ , where σ represents the root mean square of the density fluctuation of the unit cell. The model structures are shown as sticks. Carbon atoms are coloured green, yellow and purple for F. pringlei PEPC, F. trinveria PEPC and the inhibitor Asp, respectively. Nitrogen atoms are coloured blue, oxygens red and sulphurs yellow. 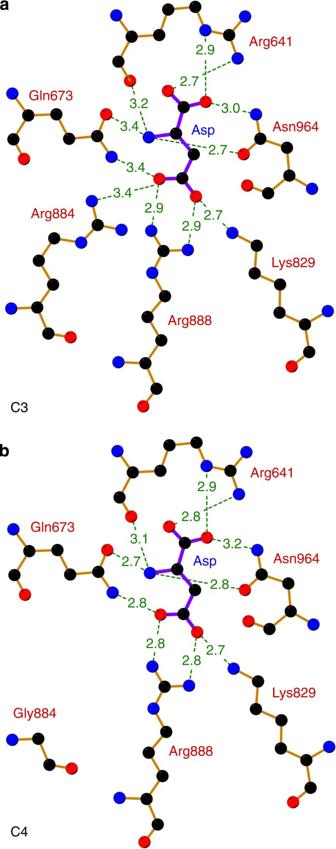Figure 4: Side by side comparison of the feedback inhibitor-binding site. (a) Inhibitor-binding site of C3 PEPC (F. pringlei). (b) Inhibitor-binding site of C4 PEPC (F. trinervia). The distances between the inhibitor aspartate and amino acids of the binding pocket are given in Å. The estimated coordinate errors are 0.24 Å (F. pringleiC3 PEPC) and 0.29 Å (F. trinerviaC4 PEPC). Residues Arg641, Lys829, Arg888 and Asn964 have been identified as the malate-binding motif15. In C3 PEPC, Arg884 provides an additional hydrogen bond for inhibitor binding. In C4 PEPC, this residue is replaced by glycine, which is 6.9 Å away from the inhibitor molecule. Full size image Figure 4: Side by side comparison of the feedback inhibitor-binding site. ( a ) Inhibitor-binding site of C3 PEPC ( F. pringlei ). ( b ) Inhibitor-binding site of C4 PEPC ( F. trinervia ). The distances between the inhibitor aspartate and amino acids of the binding pocket are given in Å. The estimated coordinate errors are 0.24 Å ( F. pringlei C3 PEPC) and 0.29 Å ( F. trinervia C4 PEPC). Residues Arg641, Lys829, Arg888 and Asn964 have been identified as the malate-binding motif [15] . In C3 PEPC, Arg884 provides an additional hydrogen bond for inhibitor binding. In C4 PEPC, this residue is replaced by glycine, which is 6.9 Å away from the inhibitor molecule. Full size image Mutagenesis and enzyme kinetics To substantiate these findings, we assessed the interactions in the malate/aspartate-binding site. We generated a series of mutations and examined their effect on the catalytic function of PEPC. When the key residue arginine 884 in C3 PEPC from F. pringlei was replaced by glycine as found in C4 PEPC, the malate tolerance of the engineered enzyme was increased by a factor of ~3. This increase corresponds to the IC 50 value obtained with C4 wild-type PEPC from F. trinervia . The reverse test is the mutation from glycine to arginine in F. trinervia C4 PEPC. This mutation resulted in an increased malate inhibition to the level of wild-type C3 PEPC from F. pringlei ( Fig. 5 ). Thus, the single aa in position 884 defines the malate-binding characteristics of the enzyme. This finding suggests that the substitution R884G is an important event in the evolution of the PEPC in the genus Flaveria . Sequence alignments with other PEPCs show that the arginine is conserved in typical C3 PEPCs while a glycine is located in the PEPCs from prominent C4 crop plants ( Fig. 6 ). These findings provide strong evidence that the substitution R884G is a key event in the evolution of a C4 PEPC in many lineages of C4 plants. 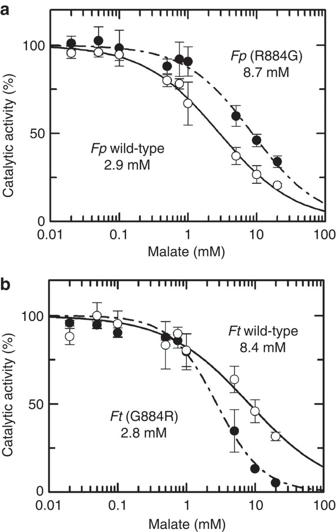Figure 5: Determination of IC50 values for wild-type and mutant PEPC fromF. pringlei(C3) andF. trinervia(C4). (a) The mean activity values ofF. pringleiwild-type C3 PEPC (open circles) andF. pringleiR884G mutant (solid circles) are plotted against the concentration of the feedback inhibitor malate. The calculated IC50values are 2.9 mM for the wild-type (solid curve) and 8.7 mM for the R884G mutant C3 PEPC (dashed curve). (b) Plot of mean activity values ofF. trinerviawild-type C4 PEPC (open circles) andF. trinerviaG884R mutant (closed circles). IC50values calculated from the experimental data are 8.4 mM for wild-type and 2.8 mM for the mutant C4 PEPC. S.d. was calculated from three independent experiments. Activities were measured in triplicates for each experiment. Figure 5: Determination of IC50 values for wild-type and mutant PEPC from F. pringlei (C3) and F. trinervia (C4). ( a ) The mean activity values of F. pringlei wild-type C3 PEPC (open circles) and F. pringlei R884G mutant (solid circles) are plotted against the concentration of the feedback inhibitor malate. The calculated IC 50 values are 2.9 mM for the wild-type (solid curve) and 8.7 mM for the R884G mutant C3 PEPC (dashed curve). ( b ) Plot of mean activity values of F. trinervia wild-type C4 PEPC (open circles) and F. trinervia G884R mutant (closed circles). IC 50 values calculated from the experimental data are 8.4 mM for wild-type and 2.8 mM for the mutant C4 PEPC. S.d. was calculated from three independent experiments. Activities were measured in triplicates for each experiment. 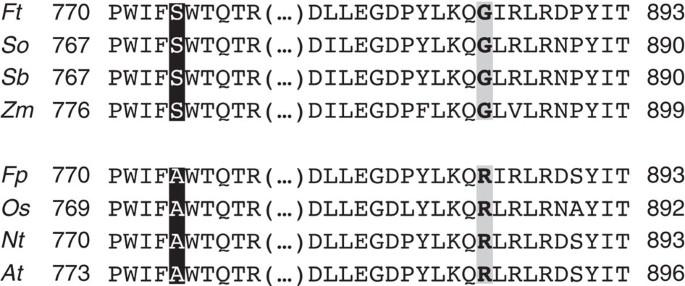Figure 6: Sequence alignment of C3 and C4 determining regions in various PEPCs. Amino acids that determine C3/C4-specific function are highlighted. In the substrate-binding centre, Ala774 (Flaverianumbering) mediates C3 specificity, while Ser774 determines the increased kinetic efficiency of C4 PEPC (black boxes). Malate binding in the inhibitory site is controlled by Arg884 in the C3 enzyme, while the increased tolerance of the C4 PEPC towards the feedback inhibitor is mediated by Gly884 (grey boxes). The sequences are:Ft(F. trinerviaUniProt No. P30694),So(Saccharum officinarumQ9FS96),Sb(Sorghum bicolorP15804),Zm (Zea maysP04711),Fp(F. pringleiGenBank CAA88829.1),Os (Oryza sativasubsp.indicaQ84XH0),Nt (Nicotiana tabacumP27154) andAt (Arabidopsis thalianaQ84VW9). Full size image Figure 6: Sequence alignment of C3 and C4 determining regions in various PEPCs. Amino acids that determine C3/C4-specific function are highlighted. In the substrate-binding centre, Ala774 ( Flaveria numbering) mediates C3 specificity, while Ser774 determines the increased kinetic efficiency of C4 PEPC (black boxes). Malate binding in the inhibitory site is controlled by Arg884 in the C3 enzyme, while the increased tolerance of the C4 PEPC towards the feedback inhibitor is mediated by Gly884 (grey boxes). The sequences are: Ft ( F. trinervia UniProt No. P30694), So ( Saccharum officinarum Q9FS96), Sb ( Sorghum bicolor P15804), Zm (Zea mays P04711), Fp ( F. pringlei GenBank CAA88829.1), Os (Oryza sativa subsp. indica Q84XH0), Nt (Nicotiana tabacum P27154) and At (Arabidopsis thaliana Q84VW9). Full size image The crystal structures of a C3-type and a C4-type PEPC obtained from two closely related species allowed us to pinpoint the molecular switch regulating feedback inhibition in a key enzyme of the C4-photosynthetic pathway. The underlying mechanism of the adapted feedback inhibitor sensitivity in C4 PEPC isoforms has not previously been identified by molecular genetics and bioinformatics. Our structural and biochemical studies reveal that the increased inhibitor tolerance is caused by a single aa substitution emphasizing that even small changes like point mutations can cause dramatic differences in kinetic and regulatory characteristics of enzymes. While residue Arg884 in the feedback inhibitor-binding pocket of C3 PEPC provides an additional hydrogen bond to the inhibitor and promotes stronger binding, the corresponding residue Gly884 in C4 PEPC reduces the steric restriction of the binding site and provides fewer contacts with the inhibitor. Therefore, the C4 enzyme is more tolerant towards feedback inhibition than the C3 enzyme. Our findings on the importance of residue 884 for malate sensitivity are not limited to the C3 and C4 species from the genus Flaveria . Alignments with other protein sequences from typical C3 and C4 PEPCs show that the arginine is conserved in C3 PEPCs, while PEPCs from typical C4 crop plants such as Z. mays , Saccharum officinarium (sugar cane) and Sorgum bicolor have a glycine at this position ( Fig. 6 ). The results show that the sensitivity of PEPC towards the feedback inhibitors malate and aspartate is accomplished by a single aa substitution at position 884. In the same way, increased PEP saturation kinetics of the C4 isoform is controlled by a single aa switch at position 774 (ref. 14 ). Nevertheless, enzymes with non-optimized feedback inhibitor-binding sites and with incomplete malate tolerance may be found in plants where high malate concentrations are circumvented by other means. For example, the PEPC of the C4-like plant Flaveria brownii carries the C4-specific aa in position 774 while an arginine remains in position 884. F. brownii is considered a C4-like species because the intercellular enzyme compartmentation is not as strict as in a true C4 plant and a substantial amount of CO 2 still enters through the C3 cycle [20] . The F. brownii PEPC therefore functions in C4-like photosynthesis but shows only moderate tolerance towards feedback inhibition [21] . The full potential of malate tolerance in such enzymes would be obtained by the glycine–arginine substitution at position 884 as realized in the C4 PEPC of F. trinvervia , though kinetic data to test this hypothesis are not available. Previous attempts to pinpoint the molecular origin of the different kinetic and regulatory characteristics of C4 PEPC suggest that multiple residues are involved in the transfer of a C3- to a C4-type enzyme [22] , [23] . Based on phylogenetic analysis of PEPC in grasses (Poaceae), Christin et al. [24] identified 21 codons that have undergone positive selection in C4 species. However, all but two of the aas concerned are identical in the C3 plant F. pringlei and the C4 plant F. trinervia. One of the C4-adaptive aa is Ser774 ( Flaveria numbering), which defines the PEP saturation kinetics [14] . The other aa is Asn659, which is—as revealed by our structural data—localized on the surface of the protein and can hardly account for the differences in inhibitor sensitivity between F. pringlei PEPC and F. trinervia PEPC. In summary, it is obvious that during evolution the main kinetic and regulatory changes of the C4 enzyme are the result of two point mutations rather than extensive modular changes such as recombination or exon shuffling. This notion is consistent with the idea that the evolution of new enzymatic activity is often achieved by the duplication of an existing gene that is capable of catalysing the chemical reaction required [22] . Within the next 50 years, the world’s population will increase by a third [25] and a corresponding increase of crop yields is needed. A concerted effort of research and development is necessary to drastically increase crop yields—similar to the ‘green revolution’ [26] . One approach is to turn C3 plants into C4 plants and, as a result, to increase the photosynthesis efficiency [27] . The best candidates for this change are the C3 plants rice and wheat, two of the most important crops of the world. Attempts were made to introduce C4 enzymes into C3 plants [28] , [29] . However, the key trigger that changes plants in anatomy as well as enzyme function and regulation has not yet been found. With our data, we complement the knowledge about PEPC, the key enzyme of C4 photosynthesis. A single mutation in the active site (774) [14] and a single mutation at the inhibitory site (884) are sufficient to switch the function from C3 to C4 activity. Now, physiological experiments could test if instead of introducing the maize PEPC into rice [28] , [29] , the rice PEPC itself could be engineered to function as a C4 enzyme. Recombinant PEPC The coding sequences of PEPC from F. trinervia (ppcA, EMBL-Bank X61304) and F. pringlei (ppcA, EMBL-Bank Z48966) were cloned in pETEV16b (Novagene), together with the coding sequence of an amino-terminal His10-tag and a TEV cleavage site. Plasmids were transformed in E. coli BL21(DE3) ( F. trinervia ) or BL21-Gold(DE3) ( F. pringlei ) (Agilent Technologies). Point mutations and truncations were introduced into the constructs as described in the QuikChange Site-Directed Mutagenesis Kit (Agilent Technologies) using Pwo polymerase. Constructs are listed in Table 2 . Cultures were grown in 2YT media (5 g l −1 sodium chloride, 10 g l −1 yeast extract and 16 g l −1 peptone) with ampicillin at 37 °C to OD 600 0.8. Production of recombinant proteins was induced with 0.5 mM IPTG and cells were grown for 18 h at 16 °C. After harvesting, cells were suspended in lysis buffer (50 mM Tris, 10 mM MgCl 2 , 150 mM NaCl, DNAse, lysozyme, pH 7.5) and disrupted by sonification. Proteins were purified by nickel affinity chromatography, concentrated by Amicon Ultra-15 centrifugal filter units (50 kDa cutoff, Millipore) and buffered in concentration buffer (50 mM Tris, 10 mM MgCl 2 , 1 mM DTT, +/− 10 mM aspartate, pH 7.5) using PD10 columns (GE Healthcare). Table 2 Constructs in pETEV16b. Full size table Crystallization Crystallization trials were performed in micro batch technique. PEPC at a concentration range of 8–10 mg ml −1 in concentration buffer was mixed with precipitation solution at a 1:1 ratio and covered with mineral oil. Precipitation solutions were 0.1 M tri-sodium citrate pH 5.6, 0.2 M ammonium sulphate and 10% (w/v) PEG 4000 ( F. pringlei ) or 15% (w/v) PEG 4000 ( F. trinervia ). After 2 days at 21 °C, crystals of a typical size of 0.5 × 0.3 × 0.3 mm 3 were obtained and transferred to cryoprotection buffer containing 32% precipitant, 48% concentration buffer and 20% ethylene glycol and swiftly cryo-cooled in liquid nitrogen. Structure determination X-ray diffraction data were collected at the European Synchrotron Radiation Facility (ESRF), Grenoble, at beamlines BM14 and ID23-2, and at EMBL/DESY, Hamburg, at beamlines DORIS X12, X13 and PETRA P14. The C3 PEPC dataset from F. pringlei was measured at 0.8726 Å wavelength (ID23-2), C3 truncated at 1.1268 Å (P14) and the C4 PEPC dataset from F. trinervia at 0.9763 Å (BM14). Data of C4 PEPC with the inhibitor aspartate were integrated with Mosflm [30] and further processed with tools of the CCP4 suite [31] , Pointless [32] and Scala [32] in particular. Initial phases of C4 PEPC ( F. trinervia ) were obtained by molecular replacement with Z. mays C4 PEPC (PDB Code: 1JQO, 73% sequence identity) using Phaser [33] . Model building was initially done automatically with ARP/wARP [34] . This step efficiently reduced model bias. Several rounds of manual building followed using Coot [35] and refinement by Refmac5 [36] using non-crystallographic restraints and partially describing the atomic displacement parameters in groups of translation, libration and screw-motion (TLS). The structure comprises two monomers within the asymmetric unit. Crystallographic symmetry completes the tetramer. Additional electron density was found at the inhibitor-binding site. However, to avoid model bias the aspartate molecule was not fitted in the structure until model building was almost complete. The structures were validated using the tools provided by Coot, CCP4 and Rampage [37] . The C3 PEPC structure from F. pringlei was obtained by essentially the same workflow. Model building started using a 3.2 Å data set collected at ERSF ID23-2. Molecular replacement was done using the C4 PEPC structure from F. trinervia . As the region comprising the His 10 -tag, the TEV protease recognition site and the first five aas of C4 PEPC were disordered in this structure, we deleted the TEV site and the first five aas (construct C3 truncated ). Crystals from this new construct C3 truncated were obtained under identical conditions and diffracted to 2.7 Å (EMBL/DESY PETRA P14). These data were integrated with XDS [38] and the model was built as described including ARP/wARP autobuilding to reduce model bias. Figures of the atomic structures were generated with Pymol (Schrödinger). Schematic diagrams of protein–ligand interactions were made using LigPlot [39] . Inhibitor studies The IC 50 of malate inhibition was determined by a coupled spectrometric assay as described [8] . In this assay, conversion of PEP to oxaloacetate is monitored via the reduction of oxaloacetate to malate by malate dehydrogenase. The reaction velocity is measured as a decrease in OD 340 resulting from the oxidation of NADH in this reaction. The inhibition of the PEPC by malate was measured in the presence of PEP (2 × K m ), at malate concentrations from 0–20 mM. The half maximal inhibitory concentrations (IC 50 ) of wild-type and mutant enzymes were calculated from the experimental data using the Grafit software package (Erithacus Software). Accession codes : Atomic coordinates and structure factors for the reported crystal structures have been deposited with the Protein Data Bank under accession codes 3zgb ( F. pringlei ) and 3zge ( F. trinervia ). How to cite this article: Paulus, J. K. et al. Greater efficiency of photosynthetic carbon fixation due to single amino-acid substitution. Nat. Commun. 4:1518 doi: 10.1038/ncomms2504 (2013).